Hyperthin nanochains composed of self-polymerizing protein shackles Protein fibrils are expected to have applications as functional nanomaterials because of their sophisticated structures; however, nanoscale ordering of the functional units of protein fibrils remains challenging. Here we design a series of self-polymerizing protein monomers, referred to as protein shackles, derived from modified recombinant subunits of pili from Streptococcus pyogenes . The monomers polymerize into nanochains through spontaneous irreversible covalent bond formation. We design the protein shackles so that their reactions can be controlled by altering redox conditions, which affect disulphide bond formation between engineered cysteine residues. The interaction between the monomers improves their polymerization reactivity and determines morphologies of the polymers. In addition, green fluorescent protein-tagged protein shackles can polymerize, indicating proteins can be stably attached to the nanochains with its functionality preserved. Furthermore we demonstrate that a molecular-recognizable nanochain binds to its partner with an enhanced binding ability in solution. These characteristics are expected to be applied for novel protein nanomaterials. Proteins self-assemble into certain structures in which the amino-acid side chains are positioned with atomic-level accuracy and held in place by numerous intramolecular interactions. Furthermore some proteins, such as actin [1] , collagen [2] and amyloid [3] , form fibrils held together by intermolecular interactions. As these sophisticated structures can be constructed without special equipment, fibrils made of either natural or artificial proteins have been studied for use in various functional materials [4] , [5] , [6] . For example, fibrils have been used as scaffolds for metals [7] , [8] and functional proteins [9] , [10] and as networks for tissue engineering applications [11] . However, the construction of highly ordered polymeric structures composed of proteins or peptides presents several difficulties. First, because the interactions between the monomers, and thus the polymerization mechanisms, are often simple, the diameters and lengths of the polymers cannot be strictly controlled by means of rational design. Second, the polymers tend to aggregate and precipitate, which hinders the construction of functional fibrils which work in solution. Third, because most protein fibrils are composed of monomers that overlap not only axially but radially, introduced modification sites of monomers inside the fibrils often destabilize their structures. Fourth, the fibrils studied to date have been relatively thick; for example, the diameters of amyloid and collagen fibrils are 5–20 nm (ref. 12 ) and 50–500 nm (ref. 13 ), respectively. If stable nanofibrils with diameters of only a few nanometres could be prepared, the resulting increase in specific surface area would increase the number of functional units, such as RGD peptide [14] and material binding peptides [15] , available for modification. One way to resolve these difficulties would be to construct a novel artificial assembly system. A protein with a pair of binding partners on opposite sides would polymerize controllably in a manner depending on the nature of the binding partners. This strategy has been used previously [16] , [17] , [18] , [19] , [20] , [21] , [22] , [23] , but there remained several problems: for example, chemical modifications of monomers to make binding sites are often necessary [16] , [17] , [18] , [19] , [20] , single strands of the polymers are supposed to break easily and to be not stable for long periods in dilute solution because they are held together by noncovalent interactions [16] , [17] , [21] , [22] , [23] , and single strands of the polymers often assemble in an uncontrolled manner [21] , [22] . In light of these difficulties, we considered a self-assembly system with monomers based on the pili of gram-positive bacteria. Pili, long filamentous protein structures that extend from bacterial surfaces [24] , form by covalent polymerization of subunits catalysed by an enzyme called sortase [25] , [26] , [27] . As pilus subunits are arranged head-to-tail, pili are thin (2–5 nm). Furthermore, they do not aggregate. Pili, including those from gram-negative bacteria, have recently attracted much attention as the inspiration for novel nanomaterials [28] , [29] , [30] . However, the biosynthesis of pili is difficult to duplicate in vitro , so we designed novel protein monomers based on the amino-acid sequence of a Streptococcus pyogenes pilus subunit (Spy0128) consisting of two domains, an N domain and a C domain [31] ( Fig. 1a ). We used a recently devised isopeptag system [32] for assembly of the monomers by means of the native intramolecular isopeptide bond in Spy0128; when Spy0128 is split into two fragments near the end of the C domain and the two fragments are then mixed together, the isopeptide bond forms irreversibly and spontaneously between them. This reaction is highly specific [32] , while enzymes such as transglutaminases catalyse isopeptide bond formation with low specificity [33] . 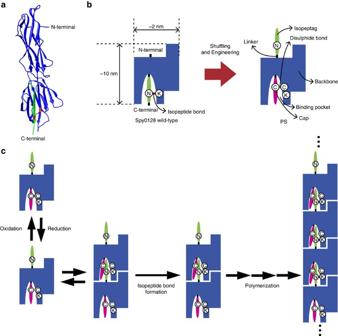Figure 1: Design of PS. (a) Crystal structure of Spy0128 (PDB 3B2M, chain B). The region corresponding to isopeptag is shown in green, and the two residues (Lys179 and Asn303) that formed an intramolecular isopeptide bond are shown in brown. The image was prepared using UCSF Chimera software. (b) Design of the PS monomer. (c) Schematic of the polymerization reaction mechanism. Figure 1: Design of PS. ( a ) Crystal structure of Spy0128 (PDB 3B2M, chain B). The region corresponding to isopeptag is shown in green, and the two residues (Lys179 and Asn303) that formed an intramolecular isopeptide bond are shown in brown. The image was prepared using UCSF Chimera software. ( b ) Design of the PS monomer. ( c ) Schematic of the polymerization reaction mechanism. Full size image Here, we devise artificial protein constructs in which the C-terminal peptide of Spy0128 (isopeptag) is transferred to the N-terminal, and the C-terminal binding pocket is protected with an engineered cap peptide that is fixed reversibly to the pocket by a disulphide bond. These protein constructs, which we refer to as protein shackles, polymerize spontaneously in a non-native head-to-tail orientation by means of an isopeptide bond between an asparagine in the N-terminal isopeptag and a conserved lysine in the C domain, which is rather analogous to the pili biosynthesis system of gram-negative bacteria [34] , [35] , [36] . The reaction is controlled by means of the redox-sensitive cap. Finally, we show that protein shackles can be functionalized by fusing any protein or peptide, indicating that they can be utilized as building blocks for high-ordered functional protein materials. Design of the PS monomer First, we constructed the PS monomer, which consisted of four main components: the isopeptag, a short linker, a backbone derived from Spy0128 and the peptide cap ( Fig. 1b and Supplementary Fig. S1 ). The native C-terminal peptide (the isopeptag) was transferred to the N-terminal and connected to the backbone via the linker, which was flexible and short enough that the N domain of one monomer could interact strongly with the C domain of the adjacent monomer. The cap was then fused to the C-terminal to prevent the artificial C-terminal binding pocket from prematurely binding to the isopeptag of another monomer. There were only three differences in sequence between the native C-terminal peptide and the cap peptide ( Supplementary Fig. S1 ): (1) the reactive asparagine of the native peptide was changed to alanine, which cannot form an intramolecular isopeptide bond; (2) the cap was shorter than the native peptide so that the cap would deviate from its resting position in the binding pocket under the polymerization conditions, and (3) most important, cysteines were introduced in both the cap and the neighbouring β strand of the backbone to permit disulphide bond formation between them. The disulphide bond formed under oxidative conditions and was cleaved under reductive conditions. Under oxidative conditions, the cap was fixed in the binding pocket, inhibiting the binding of the isopeptag of another monomer. Therefore, the polymerization reaction could be controlled simply by changing the redox conditions ( Fig. 1c ). The candidates for the cysteine mutations were calculated using the bridgeD program [37] and found to be K108C and T302C ( Supplementary Fig. S2 ). The N-terminal isopeptag of one PS monomer bound to the C-terminal binding pocket of another PS monomer only under reductive conditions, and the binding process was repeated to form a polymer ( Fig. 1c ). Reactivity and physical properties of PS We examined the reactivity of PS under oxidative and reductive conditions ( Fig. 2a ) and investigated the time course of its reaction under reductive conditions ( Fig. 2b ). Sodium dodecyl sulphate–PAGE (SDS–PAGE) analysis showed that the reactivity was greatly increased under reductive conditions, although PS reacted slightly even under oxidative conditions ( Fig. 2a ). A mutein of PS whose catalytic residue essential for the isopeptide bond formation [31] was changed to alanine, E258A, did not polymerize under either oxidative or reductive conditions ( Fig. 2a ). Furthermore another mutein whose engineered cysteines were remutated to native residues, ΔSS, polymerized under both oxidative and reductive conditions ( Fig. 2a ). These results demonstrated that the cap functioned as intended: under oxidative conditions, it was fixed to the binding pocket by the disulphide bond, and it inhibited isopeptag binding; whereas under reductive conditions, it was free to bind to the isopeptag in the binding pocket ( Fig. 1c ). Additional experiments showed that the speed of the reaction was optimal in a buffer containing dithiothreitol (DTT) at pH 9 ( Supplementary Fig. S3 ) and that the reaction could be stopped and started at will by changing the redox conditions ( Supplementary Fig. S4 ). In addition, no precipitates formed in the reaction solution, which demonstrates that the polymer was soluble in the buffer. 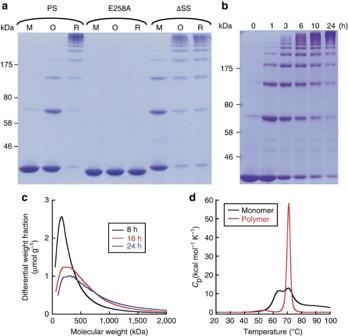Figure 2: Properties of PS. (a) Analysis of samples by 7.5% SDS–PAGE with Coomassie brilliant blue staining after 16 h of reaction. The monomers of PS, E258A and ΔSS were dissolved at concentrations of 100 μM in oxidative buffer or reductive buffer containing 5 mM DTT. M, purified monomer sample; O, reaction sample in oxidative buffer; R, reaction sample in reductive buffer. The oligomers contained in the monomer sample of ΔSS were produced during the concentration of the sample after the purification. (b) Analysis of the time course of polymerization by 7.5% SDS–PAGE with Coomassie brilliant blue staining. PS monomer was dissolved at a concentration of 100 μM in reductive buffer, and samples were analysed after 0, 1, 3, 6, 10 and 24 h of reaction. (c) Molecular weight distribution of polymer samples calculated from AF4 elution profiles. 8 h reaction sample, black; 16 h reaction sample, red; 24 h reaction sample, blue. (d) Heat capacity (Cp) curves of the monomer and the polymer measured by DSC. Monomer, black; polymer, red. Figure 2: Properties of PS. ( a ) Analysis of samples by 7.5% SDS–PAGE with Coomassie brilliant blue staining after 16 h of reaction. The monomers of PS, E258A and ΔSS were dissolved at concentrations of 100 μM in oxidative buffer or reductive buffer containing 5 mM DTT. M, purified monomer sample; O, reaction sample in oxidative buffer; R, reaction sample in reductive buffer. The oligomers contained in the monomer sample of ΔSS were produced during the concentration of the sample after the purification. ( b ) Analysis of the time course of polymerization by 7.5% SDS–PAGE with Coomassie brilliant blue staining. PS monomer was dissolved at a concentration of 100 μM in reductive buffer, and samples were analysed after 0, 1, 3, 6, 10 and 24 h of reaction. ( c ) Molecular weight distribution of polymer samples calculated from AF4 elution profiles. 8 h reaction sample, black; 16 h reaction sample, red; 24 h reaction sample, blue. ( d ) Heat capacity ( C p ) curves of the monomer and the polymer measured by DSC. Monomer, black; polymer, red. Full size image Further analysis of molecular weight distribution was carried out by asymmetric flow field flow fractionation (AF4). AF4 is a matrix-free system useful for separating molecules under mild conditions simply by changing the cross-flow rate [38] . Smaller molecules are eluted faster than larger molecules, which is the opposite of the elution order observed with size-exclusion chromatography. When an online multi-angle light-scattering detector and a transparent UV detector are attached to the AF4 system, molecular weights can be calculated continuously. In the AF4 elution profiles of polymer solutions with varied reaction time (8, 16 and 24 h) ( Supplementary Fig. S5 ), elution time became later when one with longer reaction time was analysed. This temporal change indicated that polymerization proceeded kinetically, which is consistent with SDS–PAGE analysis ( Fig. 2b ). Calculated molecular weight distribution showed broad peak ( Fig. 2c ), which suggested that this reaction exhibited the characterization of condensation polymerization. The thermostabilities of the PS monomer and polymer were measured by differential scanning calorimetry (DSC) [39] . The heat capacity change for protein denaturation was measured, and the melting temperature ( T m ), which is the temperature at the midpoint of the protein-unfolding transition, was calculated by analysing the DSC data ( Fig. 2d ). The monomer exhibited a complicated heat-capacity curve, in which the T m of the first peak appeared at about 64 °C. In contrast to the monomer, the polymer showed a simple curve, with one peak corresponding to a T m of about 71 °C, which suggests that PS was stabilized by polymerization. To determine the morphology of the polymer, we used atomic force microscopy (AFM). Mica substrates were immersed in dilute polymer solutions, dried and subsequently scanned by AFM. In the height profile of the PS polymer, many 1-nm-high C- and S-shaped nanochains were observed ( Fig. 3a–f ). These characteristic shapes might have been due to slight differences in monomer positioning between the natural Spy0128 pili and the artificial nanochains. That the curvatures of individual nanochains differed from each other indicates that they were flexible. In a magnified image of one of the nanochains ( Fig. 3g ), several knots were visible, which suggests that the nanochains were composed of tandemly aligned monomers. Considering Spy0128 crystal structure the diameters would be 2–3 nm. However, heights are prone to be underestimated by AFM [40] and there is another report that the height of single strands of some pili was measured to be <1 nm by AFM, whereas it was expected to be 3 nm considering the crystal structure [41] probably because of deformation by drying; therefore, the fibrous structures in AFM images are considered as the expected nanochains. 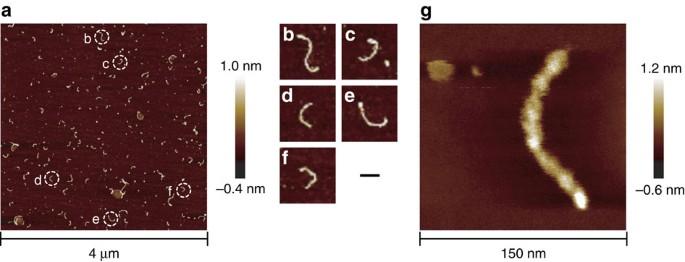Figure 3: Atomic force microscopy images of the PS polymer. (a) Height profile of the PS polymer (4 μm × 4 μm). (b–f) Magnified images of selected nanochains from (a). Scale bar, 100 nm. (g) Height profile of a nanochain (150 nm × 150 nm). Figure 3: Atomic force microscopy images of the PS polymer. ( a ) Height profile of the PS polymer (4 μm × 4 μm). ( b – f ) Magnified images of selected nanochains from ( a ). Scale bar, 100 nm. ( g ) Height profile of a nanochain (150 nm × 150 nm). Full size image Design of muteins with disrupted interaction surfaces Crystal structure analysis suggests that the N domain of one native Spy0128 subunit interacts with the C domain of the next subunit [31] ( Fig. 4a ). However, there have been no reports of interaction in solution (even when analytical ultracentrifugation was used to investigate the oligomeric state of Spy0128 (ref. 42 )), which indicates that the affinity of any interaction would have to be weaker than micromolar. 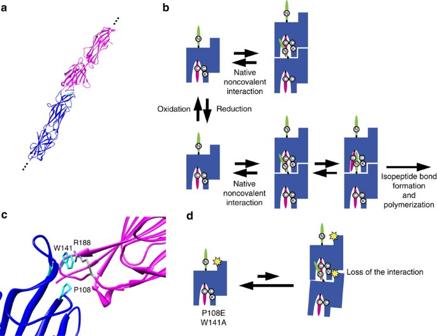Figure 4: Native noncovalent interaction between Spy0128 subunits. (a) Image of the interaction surface between Spy0128 subunits in the crystal structure (PDB 3B2M, chains B and C). Two residues that seem important for the interaction (Pro108 and Trp141) are shown in cyan; R188, which seems to interact with Trp141, is shown in grey. The image was prepared using UCSF Chimera software. (b) Detailed mechanism of PS polymerization. (c) Magnified image of the interaction surface between Spy0128 subunits in the crystal structure (PDB 3B2M, chains B and C). The image was prepared using UCSF Chimera software. (d) Design of PS muteins (P108E and W141A). The yellow star indicates the mutated residue on the interaction surface, which changed the equilibrium state of the monomer. Figure 4: Native noncovalent interaction between Spy0128 subunits. ( a ) Image of the interaction surface between Spy0128 subunits in the crystal structure (PDB 3B2M, chains B and C). Two residues that seem important for the interaction (Pro108 and Trp141) are shown in cyan; R188, which seems to interact with Trp141, is shown in grey. The image was prepared using UCSF Chimera software. ( b ) Detailed mechanism of PS polymerization. ( c ) Magnified image of the interaction surface between Spy0128 subunits in the crystal structure (PDB 3B2M, chains B and C). The image was prepared using UCSF Chimera software. ( d ) Design of PS muteins (P108E and W141A). The yellow star indicates the mutated residue on the interaction surface, which changed the equilibrium state of the monomer. Full size image We hypothesized that such an interaction might have affected our protein shackle polymerization system, because the geometries of the neighbouring monomers were similar to the native pilus. If the interaction did occur in solution, noncovalent associations might have formed before the insertion of the isopeptag into the binding pocket. We believe that noncovalently associated monomers were intermediates that lowered the activation energy of the polymerization reaction ( Fig. 4b ). To determine whether this interaction actually occurred and affected the reaction or the thermostability and morphology of the polymers, we prepared two muteins of PS (P108E and W141A; the residue numbering corresponds to the wild-type Spy0128 numbering), in which we expected the mutated residues to be essential for the interaction ( Fig. 4c,d ). Pro108 is located in the centre of the hydrophobic interaction surface, so we replaced it with glutamic acid, which has a large charged side chain, to disrupt the interaction. Trp141 forms a cation–π interaction with Arg188 of the next monomer at the edge of the interaction surface judging from the crystal structure, so we replaced it with alanine to disrupt that interaction. Reaction kinetics improved by noncovalent interaction Monomers and polymers of the muteins exhibited similar circular dichroism (CD) spectra to those of PS, suggesting that they were properly folded ( Fig. 5a ). Next, we examined the time course of the reactions of the P108E and W141A muteins under reductive conditions ( Fig. 5b ). Both muteins reacted more slowly than the PS ( Fig. 2b ). To elucidate the effect of the mutations we prepared a peptide containing an isopeptag at its N-terminal (it also contained a FLAG-tag [DYKDDDDK] followed by the N-terminal peptide of Spy0128 to give it solubility and larger molecular weight to be analysable by means of SDS–PAGE). In a competitive inhibition assay in which the polymerization was performed in the presence of a 10-fold molar excess of this peptide, PS and the two muteins showed nearly identical reactivity with the peptide ( Fig. 5c ), which indicated that the mutations did not affect the isopeptag system itself. This experiment further indicates that the binding pocket of PS reacted much more rapidly with the isopeptag of PS than that of the peptide because polymerization of PS proceeded substantially even in the presence of a 10-fold molar excess of the peptide, suggesting that the PS binding pocket recognized the isopeptag of PS with high selectivity. 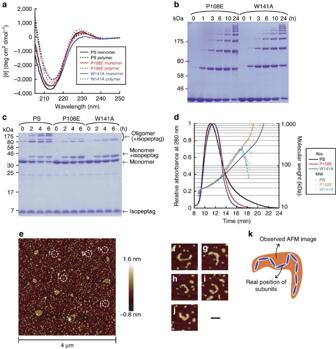Figure 5: Effects of the native noncovalent interaction. (a) The CD spectra of the monomers (solid curves) and the polymers (dashed line). PS, black; P108E, red; W141A, blue. (b) Analysis of the time course of the reactions of P108E and W141A by 7.5% SDS–PAGE with Coomassie brilliant blue staining. A 100-μM solution of each monomer in reductive buffer containing 5 mM DTT was prepared, and reaction samples were collected and analysed after 0, 1, 3, 6, 10 and 24 h. (c) Competitive polymerization inhibition assay analysed by 15% SDS–PAGE with Coomassie brilliant blue staining. Reaction solutions containing monomer (20 μM) and the isopeptag-containing peptide (200 μM, abbreviated as ‘isopeptag’ in the figure) were prepared, and reaction samples were collected and analysed after 0, 1, 3, 6, 10 and 24 h. (d) AF4 elution profiles (solid curves: PS, black; P108E, red; W141A, blue) and weight-averaged molecular weight plots (dots: PS, grey; P108E, orange; W141A, light blue) for each monomer. (e) Height profile of P108E polymer (4 μm × 4 μm). Large particle-like area is thought to be composed of remained salt or aggregated nanochains. (f–j) Magnified images of selected nanochains frome. Scale bar, 100 nm. (k) Graphical explanation of the inconsistent widths of the nanochains: (blue ellipses) protein shackle monomers making up the nanochain and (orange area) observed AFM image. Figure 5: Effects of the native noncovalent interaction. ( a ) The CD spectra of the monomers (solid curves) and the polymers (dashed line). PS, black; P108E, red; W141A, blue. ( b ) Analysis of the time course of the reactions of P108E and W141A by 7.5% SDS–PAGE with Coomassie brilliant blue staining. A 100-μM solution of each monomer in reductive buffer containing 5 mM DTT was prepared, and reaction samples were collected and analysed after 0, 1, 3, 6, 10 and 24 h. ( c ) Competitive polymerization inhibition assay analysed by 15% SDS–PAGE with Coomassie brilliant blue staining. Reaction solutions containing monomer (20 μM) and the isopeptag-containing peptide (200 μM, abbreviated as ‘isopeptag’ in the figure) were prepared, and reaction samples were collected and analysed after 0, 1, 3, 6, 10 and 24 h. ( d ) AF4 elution profiles (solid curves: PS, black; P108E, red; W141A, blue) and weight-averaged molecular weight plots (dots: PS, grey; P108E, orange; W141A, light blue) for each monomer. ( e ) Height profile of P108E polymer (4 μm × 4 μm). Large particle-like area is thought to be composed of remained salt or aggregated nanochains. ( f – j ) Magnified images of selected nanochains from e . Scale bar, 100 nm. ( k ) Graphical explanation of the inconsistent widths of the nanochains: (blue ellipses) protein shackle monomers making up the nanochain and (orange area) observed AFM image. Full size image To characterize the weakly noncovalent association in solution, we analysed the monomers in an oxidative environment by means of AF4. Recently, AF4 has been suggested as a powerful method for investigating weak protein–protein interactions ( K d >μM) in solution [43] . In the AF4 elution profiles of a PS solution ( Fig. 5d ), definite tailing with increasing weight-averaged molecular weight was observed in the UV curve, suggesting that PS formed multimers, although the beginning of the main peak corresponded to the molecular weight of the monomer (calculated to be 35 kDa). SDS–PAGE analysis showed that a polymerization reaction involved in the covalent bond formation should not have occurred in such a short time (~15 min) in an oxidative environment. Hence, the AF4 results suggest that the monomers were associated via some noncovalent interaction in solution. Analyses of the P108E and W141A muteins under the same conditions showed markedly smaller peak tailings. Therefore, we concluded that the association was largely due to noncovalent interaction between one N domain and the adjacent C domain, as mentioned above. On the basis of the combined results of kinetic analysis using SDS–PAGE and equilibrium analysis using AF4, we propose the reaction model shown in Fig. 4b . Our results indicate that even a weak interaction away from the reaction site could promote the reaction via the proximity effect. Polymer morphology determined by interaction surface Next, we used DSC and CD to measure the thermostability of the monomers and the polymers prepared from each of the three monomers ( Supplementary Figs S6,S7 ). Calculated T m and enthalpy change (Δ H VH , the van’t Hoff enthalpy change; Δ H cal , the calorimetric enthalpy change) values are summarized in Table 1 . DSC curve of each monomer did not show a simple single peak; therefore, the parameters could not be calculated. From the CD data, the P108E and W141A mutations resulted in decreases in T m of both monomers and polymers. Although the difference of T m between each monomer and polymer, Δ T m , did not show a clear trend, that of Δ H VH , ΔΔ H VH , was proved to be suppressed by the mutations, indicating that the mutated residues contributed to the specific interaction between the monomers in the polymer structure. Table 1 Thermodynamic parameters. Full size table We analysed the morphology of the polymers by means of AFM. Compared with the PS polymer, the P108E and W141A polymers ( Fig. 5e and Supplementary Fig. S8 , respectively) showed fewer distinct nanochains, which reflects their slower reactions. The nanochains of P108E did not have constant widths compared with those of PS (compare Figs 3b–f , 5f–j ), although they had similar heights of ~1 nm, suggesting that the loss of the noncovalent interaction between the monomers led to less controlled positioning of the monomers ( Fig. 5k ). Polymerization of protein shackles tagged with GFP If these polymers are to be used for functional nanomaterials, they must be functionalizable. Therefore, we genetically fused a functional protein to one terminal of PS and determined whether the fused PS could still be polymerized. We used green fluorescent protein (GFP) as the functional protein, because its fluorescence permits easy monitoring of the folding and functioning of the fused protein. GFP-PS, a PS derivative with the N-terminal linked to GFP ( Fig. 6a ), was expressed in the soluble fraction of Escherichia coli, just as the other constructs were. The purified GFP-PS monomer exhibited green fluorescence ( Supplementary Fig. S9 ), indicating that the GFP domain was correctly folded. We dissolved the fused monomer in reaction buffer containing reductant to determine whether polymerization occurred. SDS–PAGE analysis demonstrated that GFP-PS did in fact polymerize, although the reaction seemed to be slower than the reaction of PS, whereas E258A mutation resulted in a complete loss of polymerizability ( Fig. 6b,c ). Even after polymerization, the shapes of the fluorescence excitation and emission spectra were remained unchanged ( Supplementary Fig. S9 ). To quantify the loss-of-function caused by the polymerization, the fluorescence intensities were plotted versus the concentrations of GFP subunit using the monomer and the polymer of GFP–PS along with GFP as a control ( Fig. 6d ). Slopes of the plots were almost the same between them (GFP, 79.5 μM −1 , R 2 =0.994; GFP-PS monomer, 85.5 μM −1 , R 2 =0.997; GFP-PS polymer, 89.3 μM −1 , R 2 =0.997), indicating that GFP could be attached to the nanochains without disrupting their structure or function. 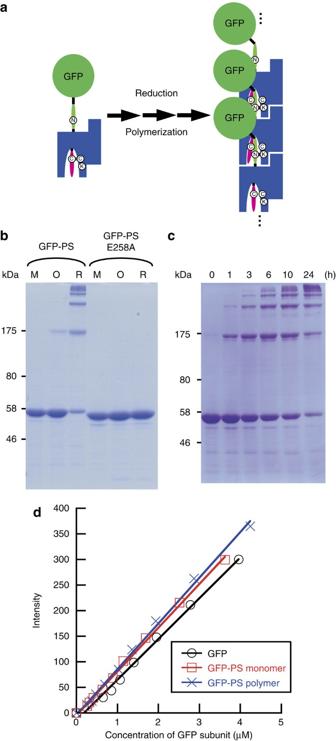Figure 6: Design and properties of GFP-PS. (a) Schematic illustration of GFP-PS design and expected polymerization reaction. (b) Analysis of the reaction sample by 7.5% SDS–PAGE with Coomassie brilliant blue staining. The monomers of GFP-PS and GFP-PS E258A were dissolved at concentrations of 100 μM in the oxidative buffer or the reductive buffer containing 5 mM DTT and allowed to polymerize for 16 h. M, purified monomer sample; O, reaction sample in oxidative buffer; R, reaction sample in reductive buffer. (c) Analysis of polymerization time course by 7.5% SDS–PAGE with Coomassie brilliant blue staining. The monomer was dissolved at a concentration of 100 μM in the reductive buffer, and reaction samples were analysed after polymerization for 0, 1, 3, 6, 10 and 24 h. (d) Standard curves of fluorescence at 515 nm relative to GFP subunit concentration. GFP, black circle; GFP-PS monomer, red square; GFP-PS polymer, blue cross. Figure 6: Design and properties of GFP-PS. ( a ) Schematic illustration of GFP-PS design and expected polymerization reaction. ( b ) Analysis of the reaction sample by 7.5% SDS–PAGE with Coomassie brilliant blue staining. The monomers of GFP-PS and GFP-PS E258A were dissolved at concentrations of 100 μM in the oxidative buffer or the reductive buffer containing 5 mM DTT and allowed to polymerize for 16 h. M, purified monomer sample; O, reaction sample in oxidative buffer; R, reaction sample in reductive buffer. ( c ) Analysis of polymerization time course by 7.5% SDS–PAGE with Coomassie brilliant blue staining. The monomer was dissolved at a concentration of 100 μM in the reductive buffer, and reaction samples were analysed after polymerization for 0, 1, 3, 6, 10 and 24 h. ( d ) Standard curves of fluorescence at 515 nm relative to GFP subunit concentration. GFP, black circle; GFP-PS monomer, red square; GFP-PS polymer, blue cross. Full size image Function of nanochain fused low-affinity peptide binders As an example of an application of the soluble nanochain composed of protein shackles, we used functionalized nanochains as a novel type of ‘antibody’. Immunoglobulin is known to have multiple antigen-binding sites, which improves its binding ability, This phenomenon is called avidity effect [44] . Therefore, a polymer composed of monomers, which have weak but specific binders, is expected to have an enhanced binding property. We chose a pair of peptides named VAAL K3 and VAAL E3 as a model interaction system [45] . They are composed of 21 residues and form a coiled-coil heterodimer with an affinity ( K D ) of 4 μM (ref. 45 ). K3-PS, a PS derivative with the N-terminal linked to VAAL K3, was prepared as an ‘antibody’, whereas GST-E3, VAAL E3 tagged with a His 6 and a glutathione S-transferase (GST) in its N-terminal, was prepared as an ‘antigen’. Surface plasmon resonance (SPR) was employed to characterize their interactions. Sample solutions containing K3-PS monomers or polymers were injected into a sensor chip where GST-E3 had been immobilized ( Fig. 7a ). We used two polymer samples with different reaction times (3 and 16 h) ( Fig. 7b ). Real-time response curves when 31.3 nM (monomer concentration) of the samples were analysed are shown in Fig. 7c . In this condition, 16 h reaction sample had the best binding ability (5.1-fold binding level at 180 s compared with the monomer). To analyse the concentration dependency on the binding ability, normalized responses at 180 s were plotted at different concentrations ( Fig. 7d ). This plot suggested that an initial rise of the response started at lower concentration when using K3-PS with higher degrees of polymerization. Thus, our molecular-recognizable nanochain has achieved a high-binding ability to the target by polymerization. 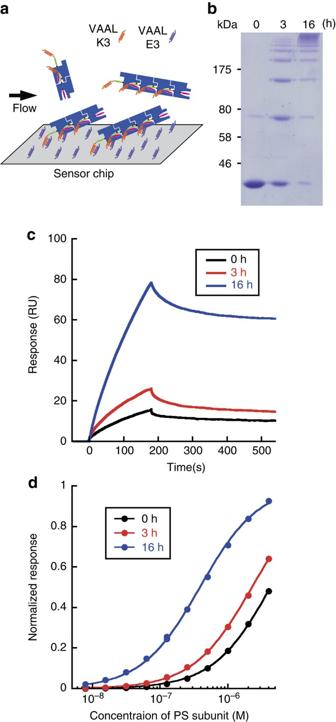Figure 7: Interaction analysis of K3-PS polymer. (a) Schematic image of the experiment. GST-E3 was immobilized in a sensor chip through His6-tag and then the monomer or the polymer solution of K3-PS was injected. SPR response from binding of K3-PS to the chip was monitored. (b) Analysis of the injected sample by 7.5% SDS–PAGE with Coomassie brilliant blue staining. Monomer (0 h) was dissolved at a concentration of 100 μM in reductive buffer, and samples were analysed after polymerization for 3, 16 h. (c) Sensorgram of each sample at a monomer concentration of 31.3 nM. Zero hour reaction sample (monomer), black; 3 h reaction sample, red; 16 h reaction sample, blue. (d) Binding level plot at 180 s normalized byRmaxcalculated from the curve fitting relative to the monomer concentration of K3-PS. Zero hour reaction sample (monomer), black; 3 h reaction sample, red; 16 h reaction sample, blue. Figure 7: Interaction analysis of K3-PS polymer. ( a ) Schematic image of the experiment. GST-E3 was immobilized in a sensor chip through His 6 -tag and then the monomer or the polymer solution of K3-PS was injected. SPR response from binding of K3-PS to the chip was monitored. ( b ) Analysis of the injected sample by 7.5% SDS–PAGE with Coomassie brilliant blue staining. Monomer (0 h) was dissolved at a concentration of 100 μM in reductive buffer, and samples were analysed after polymerization for 3, 16 h. ( c ) Sensorgram of each sample at a monomer concentration of 31.3 nM. Zero hour reaction sample (monomer), black; 3 h reaction sample, red; 16 h reaction sample, blue. ( d ) Binding level plot at 180 s normalized by R max calculated from the curve fitting relative to the monomer concentration of K3-PS. Zero hour reaction sample (monomer), black; 3 h reaction sample, red; 16 h reaction sample, blue. Full size image We expected the diameters of the nanochains to be 2–3 nm in solution, and the measured diameters were as small as 1 nm when measured in air by AFM, which is much smaller than the diameters of typical protein fibrils. We attributed this hyperthinness to the covalent cross-linkage between the monomers. The sum of noncovalent interactions in such a small cross-section alone would not be sufficient to allow stable axial elongation of the fibril, which may be one of the reasons that the native pili of gram-positive bacteria also rely on covalent cross-linkages between subunits but in a different form than in our system [25] , [26] , [27] . One of the advantages of the smaller diameter is the larger specific surface area, which enables the chain to present more functionalizable sites per unit volume. This means the characteristics of the nanochain can be readily tuned by the addition of modifying molecules. Here, we constructed a GFP-PS polymer. As GFP has a molecular weight of 26 kDa and that of PS is 35 kDa, the GFP domains, which were fully presented to the solvent, accounted for over 40% of the GFP-PS polymer. Another advantage of this nanochain as a novel functional material is its ~10 nm periodicity. In a previous study in which amyloidogenic peptides tagged with yellow fluorescent protein were polymerized to form amyloid fibrils, most of the fluorescence was lost upon polymerization [46] , which suggests that the yellow fluorescent protein domains denature due to their dense packing. In our case, the GFP domains were positioned along the nanochain at ~10-nm intervals, which allowed the GFP domains to retain their fluorescence after the GFP-PS was polymerized. Although reports indicate that some protein fibrils can present short peptides with nanoscale periodicity [8] , [47] , it is unclear whether large functional proteins can be fused to those fibrils, because modification with proteins often destabilizes such assemblies. Hence, the fact that large functional proteins could be axially spaced at 10-nm intervals is a unique strong point of our nanochains. Finally, we demonstrated that the nanochain functionalized by the molecular-recognizable peptide functioned effectively in solution. As protein shackles with other functionalities can be prepared easily, multifunctional nanochains will be synthesized by copolymerization of protein shackles with different functions such as an antibody and an enzyme. In conclusion, we engineered novel protein monomers, referred to as protein shackles, which polymerized via spontaneous covalent bond formation to form soluble hyperthin nanochains. The polymerization reaction could be controlled by changing the redox conditions, which affected the engineered disulphide bond of the cap fixed reversibly to the binding pocket. In addition, our results suggest that weak noncovalent interactions between the monomers facilitated the polymerization reaction and affected the morphologies of the polymers. Furthermore, GFP-tagged protein shackles polymerized without loss of the fluorescence of GFP. Also a molecular-recognizable peptide was proved to be enhanced its binding ability simply by fusing to a nanochain made of protein shackles. We expect that our protein shackles will be useful for the preparation of various highly ordered materials including detection reagents, tunable hydrogels and organic–inorganic nanocomposites, depending on whether the nanochains are modified with a small-molecule, a short peptide, a functional protein or their combinations. Preparation of protein shackles Detailed procedures for cloning, expression and purification are described in Supplementary Methods . In brief, proteins were expressed in E. coli BL21 (DE3) cells transformed with pCold II vectors (Takara Bio) into which the target nucleotide sequences had been inserted. The monomers were purified from cell lysates by immobilized metal affinity chromatography and gel-filtration chromatography. Protein concentrations were determined spectrophotometrically at 280 nm from the calculated molar extinction coefficients of the proteins. The identity of the purified monomers was verified by matrix-assisted laser desorption ionization mass spectrometry (see Supplementary Methods ). The proteins were frozen in liquid nitrogen and stored at −30 °C. Preparation of monomers for polymerization reaction Monomers were precipitated from solution with acetone, and the precipitates were dried in a vacuum desiccator for about 15 min. Dried powders were dissolved in a given amount of the reaction buffer (50 mM glycine-NaOH and 5 mM DTT typically at pH 9.0); the time of dissolution was defined as the start time of the reaction. All the reactions described in this paper were done at room temperature. Sodium dodecyl sulphate–polyacrylamide gel electrophoresis Samples were prepared as mixed solutions of 5 μl of about 1.5 mg ml −1 protein solution, 12 μl of sample buffer (80 mM sodium dodecyl sulphate, 62.5 mM Tris–HCl, 8% glycerol; pH 6.8 at room temperature), 2 μl of 1 mg ml −1 bromophenol blue solution containing 10% glycerol and 1 μl of 2-mercaptoethanol, then boiled for 5 min. The samples were loaded onto a polyacrylamide gel containing 0.1% sodium dodecyl sulphate. Electrophoresis was performed at 150 V for 70–90 min. Gels were stained with 0.5% Coomassie brilliant blue R-250. Asymmetrical flow field flow fractionation Protein association was analysed by AF4 with a Wyatt Eclipse separation system (Wyatt). The instrument was equipped with UV–visible and multi-angle light-scattering detectors, and a cellulose membrane with a nominal molecular weight cutoff of 5 kDa was used for separation. For analysing polymer solution, samples were concentrated with a focus flow (flow rate 1.5 ml min −1 ) and then eluted with a cross flow decreased linearly from 1.5 to 0.5 ml min −1 over the course of the first 5 min, from 0.5 to 0.2 ml min −1 over the course of the next 5 min, and from 0.2 to 0.0 ml min −1 over the course of the last 10 min. For analysing monomer solution, samples were concentrated with a focus flow (flow rate 3.0 ml min −1 ) and then eluted with a cross flow held at 3.0 ml min −1 for 2 min and then decreased linearly from 3.0 to 0.0 ml min −1 over the course of 15 min. The channel flow rate was maintained at 1.0 ml min −1 . Each experiment required about 200 μg of protein. Phosphate buffered saline (PBS; 137 mM NaCl, 2.7 mM KCl, 10 mM Na 2 HPO 4 , 1.8 mM KH 2 PO 4 , pH 7.4) was used for the mobile phase buffer. Molecular weights were determined from the multi-angle light-scattering data and Zimm plot analysis by means of the ASTRA software package (Wyatt) provided with the instrument. Each molecular weight distribution was calculated from a main peak of the elution profile (8 h reaction sample, from 7.5 to 12.0 min; 16 h reaction sample, from 8.0 to 15 min; 24 h reaction sample, from 8.0 to 15.5 min) by means of the ASTRA software. Differential scanning calorimetry Heat capacity curves were measured on a VP-DSC ultrasensitive scanning calorimeter (MicroCal). A solution of each monomer (100 μM) in a buffer containing 50 mM glycine-NaOH and 5 mM DTT at pH 9.0 was allowed to react for 16 h (PS) or 48 h (P108E, W141A, P108E and W141A) to form the corresponding polymer sample. Monomer and polymer samples were prepared at a monomer concentration of about 25 μM in PBS. The scan rate was 1 K min −1 . Data were analysed with the ORIGIN software package (MicroCal). To obtain the thermodynamic parameters T m and Δ H cal , we subtracted the contribution of the buffer, normalized by the protein concentration and fitted the data to a two-state thermal transition model. CD spectroscopy The CD spectroscopy experiments were measured on a JASCO J-820 CD spectrometer (JASCO). The preparation method of the polymers was the same as described in the section of DSC above. The proteins were used at a concentration of 0.25 mg ml −1 in PBS. Two-millimetre path length quartz cuvette was used. Spectra were collected at 20 °C (resolution; 0.1 nm, average time; 4 s, scan speed; 200 nm min −1 ) and obtained by taking the average of four scans made from 250 to 205 nm. For thermal melting, temperature was increased from 20 to 90 °C at a rate of 1 K min −1 and signals at 222 nm were collected at 0.1 K intervals. The obtained thermal denaturation curves were fitted to a two-state transition model by a JASCO software to obtain the thermodynamic parameters T m and Δ H VH . Atomic force microscopy Morphology was observed by means of AFM with a MultiMode 8 system (Bruker). A solution of each monomer (200 μM) in a buffer containing 50 mM glycine-NaOH and 5 mM DTT at pH 9.0 was allowed to react for 5 days to form the corresponding polymer sample. Each polymer sample was diluted to a monomer concentration of about 10 nM with 50 mM Tris-HCl (pH 8.0), and the diluted sample was loaded onto a mica substrate. After 5 min, the solution was removed with a nitrogen flow. The substrate was washed a few times with Milli-Q water and then dried with a nitrogen flow. The dried mica substrate was scanned in the microscope’s ScanAsyst mode. Fluorescence assay The fluorescence intensities of GFP and GFP-PS were monitored in a quartz cuvette (path length; 1 cm, path width; 2 mm) with a spectrofluorometer F-2500 (Hitachi). The excitation wavelength was set at 500 nm and fluorescence intensities at 515 nm were monitored. Data were collected at room temperature and obtained by taking the average of three scans. A polymer sample was prepared from GFP-PS monomer (100 μM) in a buffer containing 50 mM glycine-NaOH and 5 mM DTT at pH 9.0 and reacted for 24 h. Each sample was diluted with PBS. Surface plasmon resonance SPR was employed to analyse the interaction between VAAL E3 and VAAL K3 in a Biacore T200 instrument using a sensor chip NTA (GE Healthcare). GST-E3 was immobilized at a level of about 2000 RU at the beginning of every run cycle. Each run consisted of consecutive injections of analyte (K3-PS) in a sensor chip in a buffer composed of 10 mM HEPES, 150 mM NaCl, 50 μM EDTA, 4 mM imidazole, 0.05% Tween 20 at pH 7.4, at a flow rate of 30 μl min −1 . Imidazole was added to the buffer in order to reduce a nonspecific interaction between K3-PS and nitrilotriacetic acid (NTA). The flow-cells were regenerated with a buffer composed of 10 mM HEPES, 150 mM NaCl, 0.35 M EDTA, 0.05% Tween 20 at pH 8.3 followed by 50 mM NaOH. The data were corrected by subtracting the responses from a blank flow-cell in which Ni 2+ was charged to NTA and then the responses from a flow-cell in which GST-E3 was captured when 0 M analytes were analysed. Responses at 180 s were ploted against concentrations of PS subunit, then fitted by equation: where R is the SPR response at 180 s, R max is the estimated maximum response, K A is the association constant, and C is the concentration of PS subunit. SPR data were analysed with the Biacore T200 Evaluation software (GE Healthcare). How to cite this article: Matsunaga, R. et al. Hyperthin nanochains composed of self-polymerizing protein shackles. Nat. Commun. 4:2211 doi: 10.1038/ncomms3211 (2013).